The stability of P2-layered sodium transition metal oxides in ambient atmospheres Air-stability is one of the most important considerations for the practical application of electrode materials in energy-harvesting/storage devices, ranging from solar cells to rechargeable batteries. The promising P2-layered sodium transition metal oxides (P2-Na x TmO 2 ) often suffer from structural/chemical transformations when contacted with moist air. However, these elaborate transitions and the evaluation rules towards air-stable P2-Na x TmO 2 have not yet been clearly elucidated. Herein, taking P2-Na 0.67 MnO 2 and P2-Na 0.67 Ni 0.33 Mn 0.67 O 2 as key examples, we unveil the comprehensive structural/chemical degradation mechanisms of P2-Na x TmO 2 in different ambient atmospheres by using various microscopic/spectroscopic characterizations and first-principle calculations. The extent of bulk structural/chemical transformation of P2-Na x TmO 2 is determined by the amount of extracted Na + , which is mainly compensated by Na + /H + exchange. By expanding our study to a series of Mn-based oxides, we reveal that the air-stability of P2-Na x TmO 2 is highly related to their oxidation features in the first charge process and further propose a practical evaluating rule associated with redox couples for air-stable Na x TmO 2 cathodes. Practical application is always the ultimate goal for state-of-the-art technologies and devices, such as perovskite solar cells, thin-film transistors, and electrochemical batteries [1] . Air-stability is undeniably one of the key issues that researchers should consider, because any air-instable compounds must be prepared, stored and assembled in dry or even inert atmospheres, leading to an increase in expense and can even jeopardize whether they are successfully commercialized. Sodium ion batteries (SIBs) promise the potential for large-scale grid storage, due to the high abundance and wide distribution of Na sources as compared to their lithium counterparts [2] , [3] , [4] . Among various sodium storage cathodes, layered sodium transition metal oxides (Na x TmO 2 ) have gained significant attention owing to their great variety of compositions, ease of scalable preparation and high reversible specific capacity [5] . In the past forty years [6] , [7] , the Na x TmO 2 family has been greatly enriched not only thanks to the tremendous efforts toward superior cathodes with higher energy density and more stable structures [8] , [9] , [10] , but has also benefited from the development of electrolytes and characterization techniques [11] , [12] , [13] , [14] . Nonetheless, Na x TmO 2 electrodes are still haunted by three major challenges, i.e. irreversible phase transitions during cycling, insufficient electrochemical performances and air/moisture instability [5] , [15] . The undesired structural transformations in charge/discharge processes, such as P2-O2 in Na 0.67 Ni 0.33 Mn 0.67 O 2 [16] , [17] , [18] , [19] , [20] , P2-P2’ in Na 0.67 MnO 2 [10] , [21] , [22] , [23] and O3-P3 in NaNi 0.5 Mn 0.5 O 2 [24] , can be suppressed or delayed by element substitution, thus resulting in improved cycling stability and rate capability. The contact between air-instable Na x TmO 2 and moisture-air usually produces cracks [25] , electrical insulation species [26] , and hydration phases [27] , which result in a shorter lifetime and poorer rate capability of the exposed layered oxides [28] , [29] , [30] . Therefore, air-stability is considered an important factor to evaluate a qualified Na x TmO 2 electrode [31] , [32] , [33] . Recently, Manthiram’s group reported that O3-NaNi 0.7 Mn 0.15 Co 0.15 O 2 reacts with H 2 O and CO 2 , generating NaOH, Na 2 CO 3 , Na 2 CO 3 ∙H 2 O and NiO on the particle surfaces and leading to declined electrochemical performances [26] . However, these degradation (Ni loss) reactions have not yet been extensively observed in Ni-poor/Ni-free Na x TmO 2 materials, whether exposed to air or immersed in water [34] , [35] . Unlike degradation, H 2 O insertion is widely encountered in P2-Na x TmO 2 electrodes and can be easily distinguished by X-ray diffraction (XRD), because the intercalation of H 2 O expands the interlayer distance of the Na + layers from ~5 to ~7 Å and even up to ~9 Å [36] , [37] , [38] . Kubota et al. proposed the Na + /H + exchange mechanisms in O3-type NaMeO 2 oxides [39] and Rojo’s group further identified the presence of H + in the Na + layers using a neutron powder diffraction technique [30] . In addition, in the presence of H 2 O, CO 2 was believed to get inserted into the transition metal layers of P2-Na 2/3 Fe 0.5 Mn 0.5 O 2 [28] . These works provide valuable insights into the structural evolutions of Na x TmO 2 upon air-exposure. However, rational connections between these intertwined reactions, especially as to why and when the water molecules insert into the Na + layers, and which factor determines the extent of the structural transformation have not been thoroughly studied yet. Fundamental understanding of structural/chemical evolutions in moisture is not only critical for the employment of Na x TmO 2 as electrodes in both organic and aqueous SIBs, but also provides guidance to the fabrication and application of layered transition metal oxides in other battery systems, such as the favorable Ni-rich [40] , [41] , [42] , [43] cathodes for lithium ion batteries. For layered sodium-based oxides, it is widely recognized that the air-instability in P2-type oxides is much more severe than that in O3-type Na x MnO 2 [5] . Herein, based on the P2-Na 0.67 MnO 2 and P2-Na 0.67 Ni 0.33 Mn 0.67 O 2 oxides, we unearth the underlying science that triggers the hydration of P2-Na x TmO 2 , apply unique solid-state nuclear magnetic resonance techniques (ss-NMR) to provide solid evidence for H + insertion, analyze critical factors that influence the hydration, and outline the structural and chemical evolution mechanisms of P2-Na x TmO 2 oxides upon air exposure. Importantly, the surface-sensitive time-of-flight secondary ion mass spectroscopy (TOF-SIMS) results reveal that the CO 2 cannot insert into the layered structure. Our results indicate that Na + /H + exchange, rather than O 2 oxidation, dominates the compensation of extracted Na + and the hydration is closely related to the contents of remaining Na + ions in the structure. The critical sodium content n c is therefore proposed to evaluate whether H 2 O is able to intercalate into the sodium layers. In addition, the study of a series of P2-Na x TmO 2 oxides indicates that the air-stability is closely associated with the voltage features of the charge process in the first cycle, and a practical principle related to the redox couple in the 1 st cycle is thus proposed to evaluate the air-stability of Na x TmO 2 . These new insights into the degradation mechanisms upon air-exposure will facilitate the development of practical layered Li/Na/K transition metal oxides. Features of hydration phases To investigate the air-stable mechanisms, the structures and characterizations of hydration phases should be clarified first. The Na 0.67 MnO 2 sample attained by solid-state reaction exhibits a typical P2 structure (space group: P6 3 /mmc ) with a layer spacing of ~5.5 Å (Fig. 1 ), according to the powder X-ray diffraction (XRD) patterns in Supplementary Fig. 1a . The commonly reported hydration impurity phase in the Na x TmO 2 is birnessite [27] , [30] , [37] , whose structure is very similar to that of P2-Na 0.67 MnO 2 , except the presence of extra water molecules in the sodium layers and a broader interlayer distance of ~7.1 Å. With further H 2 O insertion, the buserite phase with layer spacing of ~9.1 Å can be identified (Fig. 1 and Supplementary Fig. 1a ). In addition to the difference in the interlayer spacing, the birnessite and buserite phases possess a different pattern of Na + and H 2 O arrangements in the sodium layers. 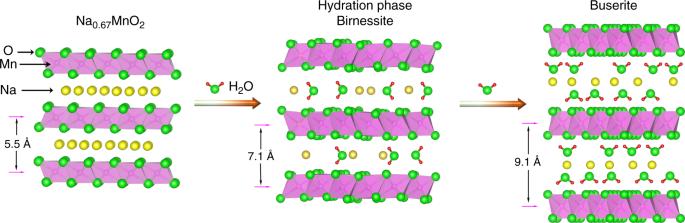Fig. 1: Structural illustration of water insertion. Schematic illustration of P2-Na0.67MnO2, birnessite, and buserite phases. For birnessite ({Na 0.30 •(H 2 O) 0.45 }MnO 2 ), according to the Rietveld refinement results [44] (Supplementary Table 1 and Fig. 1b ) and the neutron powder diffraction patterns (NPD) [45] , the O ion of inserted H 2 O molecule locates at the same site of Na + ; while for the highly hydrated buserite ({Na 0.24 •(H 2 O) 2.1 }MnO 2 ), the Na + ions are sandwiched by the inserted H 2 O molecules [46] , [47] , as illustrated schematically in Fig. 1 . Since buserite is seldom encountered in the moisture-exposed Na x TmO 2 , the hydration phase discussed below is referred to birnessite phase unless otherwise specified. It should be further pointed out that the Na + content in hydrated Na 0.67 TmO 2 sample is <0.67 due to the Na + loss upon air-exposure, as shown in the following sections. XRD, NPD and 23 Na magic-angle-spinning nuclear magnetic resonance spectroscopy (MAS NMR, Supplementary Figs. 1 – 3 and Note 1 ) are three powerful techniques to identify the hydration impurities (birnessite) in Na x TmO 2 oxides, by characterizing the structural transitions, i.e. increased interlayer spacings. Fourier-transform infrared spectroscopy (FTIR) and 23 Na{ 1 H} rotational-echo double-resonance (REDOR) [48] can be used to detect the existence of water molecules and protons in the Na x TmO 2 compounds, respectively (Supplementary Fig. 4 and Notes 1 , and 2 ). Fig. 1: Structural illustration of water insertion. Schematic illustration of P2-Na 0.67 MnO 2 , birnessite, and buserite phases. Full size image The structural transitions of the moisture-exposed P2-Na 0.67 TmO 2 To investigate the structural changes of P2-Na x TmO 2 during the air-exposure, Na 0.67 MnO 2 and Na 0.67 Ni 0.33 Mn 0.67 O 2 were selected as model compounds for air-instable and air-stable electrodes, respectively [27] , to be exposed in different atmospheres of dry CO 2 , relative humidity (RH) 18% (without CO 2 ), RH 15% + CO 2 (with presence of CO 2 ), and RH 93% + CO 2 for 3 days (“Methods” part). As shown in the XRD patterns (Fig. 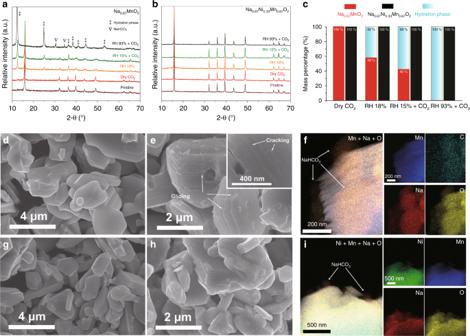Fig. 2: The structural transitions of P2-Na0.67TmO2upon air-exposure. The XRD patterns ofaNa0.67MnO2andbNa0.67Ni0.33Mn0.67O2samples exposed in different atmosphere.cThe refinement results of exposed Na0.67MnO2and Na0.67Ni0.33Mn0.67O2samples with a two-phase model. The SEM images ofdpristine andeRH 93% + CO2exposed Na0.67MnO2powder,fThe EDS mapping results of exposed Na0.67MnO2, indicating that NaHCO3is formed on the particles’ surface. The SEM images ofgpristine andhRH 93% + CO2exposed Na0.67Ni0.33Mn0.67O2powder.iThe EDS mapping results of RH 93% + CO2exposed Na0.67Ni0.33Mn0.67O2samples, NaHCO3particles are also observed on the surface of exposed Na0.67Ni0.33Mn0.67O2. The exposure time of the above samples are 3 days. 2a, b ) and inductively coupled plasma-atomic emission spectrometry (ICP-AES) results (Supplementary Table 2 ), the targeted materials were successfully prepared. It can be observed that all XRD peaks of Na 0.67 MnO 2 remain unchanged when placed in the dry CO 2 atmosphere (Fig. 2a ), revealing that water is an inevitable component to destabilize Na 0.67 TmO 2 . At the atmospheres of RH 18% and RH 15% + CO 2 , the hydration peaks (labeled with ‡) emerge and their intensities increase with the presence of CO 2 . With further increase in the relative humidity (RH 93% + CO 2 ), all of the XRD peaks can be indexed to the hydration phase and NaHCO 3 (labeled with ∇ ), indicating that the Na 0.67 MnO 2 is totally hydrated and partial Na + diffuses out from the sodium layers. For Na 0.67 Ni 0.33 Mn 0.67 O 2 , no obvious hydration peaks can be identified in all of the exposed samples (Fig. 2b ), suggesting Na 0.67 Ni 0.33 Mn 0.67 O 2 is more stable than Na 0.67 MnO 2 in moist atmospheres. To quantify the hydration extent of the exposed samples, Rietveld refinements on the XRD patterns were conducted with a two-phase model and the results are shown in Fig. 2c . The mass ratios of hydrated phases in the exposed Na 0.67 MnO 2 samples are 0%, 42%, 58%, and 100% at the atmosphere of dry CO 2 , RH 18%, RH 15% + CO 2 , and RH 93% + CO 2 , respectively, revealing that P2-Na x TmO 2 components are more vulnerable to H 2 O with both the existence of CO 2 and the increment of relative humidity. Fig. 2: The structural transitions of P2-Na 0.67 TmO 2 upon air-exposure. The XRD patterns of a Na 0.67 MnO 2 and b Na 0.67 Ni 0.33 Mn 0.67 O 2 samples exposed in different atmosphere. c The refinement results of exposed Na 0.67 MnO 2 and Na 0.67 Ni 0.33 Mn 0.67 O 2 samples with a two-phase model. The SEM images of d pristine and e RH 93% + CO 2 exposed Na 0.67 MnO 2 powder, f The EDS mapping results of exposed Na 0.67 MnO 2 , indicating that NaHCO 3 is formed on the particles’ surface. The SEM images of g pristine and h RH 93% + CO 2 exposed Na 0.67 Ni 0.33 Mn 0.67 O 2 powder. i The EDS mapping results of RH 93% + CO 2 exposed Na 0.67 Ni 0.33 Mn 0.67 O 2 samples, NaHCO 3 particles are also observed on the surface of exposed Na 0.67 Ni 0.33 Mn 0.67 O 2 . The exposure time of the above samples are 3 days. Full size image Figure 2d–i depicts the morphological change of Na 0.67 MnO 2 and Na 0.67 Ni 0.33 Mn 0.67 O 2 powder after the exposure to the atmosphere of RH 93% +  CO 2 for 3 days. Scanning electron microscopy (SEM) images in Fig. 2d, g show that the surface of as-prepared Na 0.67 MnO 2 and Na 0.67 Ni 0.33 Mn 0.67 O 2 particles are clean and smooth. After exposure, severe delamination damages and a massive of intragranular cracks can be observed in hydrated Na 0.67 MnO 2 sample (Fig. 2e ), as a result of the significant volume expansion of ~30% during the hydration process. Besides structural changes, NaHCO 3 particles are found on the surface of hydrated Na 0.67 MnO 2 , as shown in the energy dispersive X-ray spectroscopy (EDS) elemental mapping results (Fig. 2f ). Moreover, the crystals with very regular morphologies can be observed in the exposed-Na 0.67 MnO 2 powder (Supplementary Fig. 5a, b ), which should be unambiguously identified to NaHCO 3 , according to the FTIR (Supplementary Fig. 4a ) and EDS mapping results in Supplementary Fig. 5c . The formation of sodium salt is also observed in the air-exposed electrodes. As shown in Supplementary Fig. 6 , sodium bicarbonate particles with nanoflakes morphology appear at the surface of the active materials. For exposed-Na 0.67 Ni 0.33 Mn 0.67 O 2 sample, as shown in Fig. 2h , a rough surface is formed and there is no evidence of crack and layer glide, indicating that the morphological change of Na 0.67 Ni 0.33 Mn 0.67 O 2 during exposure is more moderate than the Na 0.67 MnO 2 sample (Fig. 2e ). However, the EDS mapping results in Fig. 2i reveal that the NaHCO 3 particles are formed on the surface of exposed Na 0.67 Ni 0.33 Mn 0.67 O 2 , indicating the Na + loss in Na 0.67 Ni 0.33 Mn 0.67 O 2 compound during exposure. In summary, the above XRD, SEM and EDS results indicate that Na 0.67 MnO 2 samples experience chemical transitions upon air-exposure, and Na 0.67 Ni 0.33 Mn 0.67 O 2 changes as well. Several influential factors especially relative humidity must be taken into consideration during the air-exposure experiments, soaking the samples in water is therefore a widely accepted testing procedure for confirming the stability of layered Na x TmO 2 oxides [31] . Moreover, water-stability is an important metric of Na x TmO 2 when applied as aqueous battery electrodes. Therefore, the structural evolutions of Na 0.67 MnO 2 and Na 0.67 Ni 0.33 Mn 0.67 O 2 samples in water have also been investigated. The results in Supplementary Figs. 7 and 8 and detailed analysis in Supplementary Note 3 suggest that the structural transformation mechanisms of P2-Na x TmO 2 in water are similar to that in moist air. The role of CO 2 The presence of CO 2 makes a big difference in the structural transformations of P2-Na x TmO 2 upon moisture-exposure (Fig. 2c ). To characterize the functionality of CO 2 , we applied the TOF-SIMS to ascertain whether CO 2 intercalates into the bulk of the P2-Na x TmO 2 during hydration [5] , [26] , [27] , [28] , [30] . In order to eliminate the influence of the surficial sodium bicarbonate species (Fig. 2f and Supplementary Fig. 4 ), we adopted a scavenging process (see details in the Methods section). The FTIR spectra in Fig. 3a reveal that NaHCO 3 in the hydrated Na 0.67 MnO 2 sample is successfully removed. TOF-SIMS depth profiles acquired on the scavenged powder show that the H 2 O (OH − ) and Mn ions (MnO − and MnO 2 − ) appear at both surface and bulk of the powder (Fig. 3b ), in good agreement with our refinement results (Supplementary Table 1 ). The signal intensity of C 2 HO − in the bulk (~165 a.u., Supplementary Fig. 9 and Note 4 ) is only 2.5 ‰ compared to that of the prevailed OH − (65k a.u.). Considering that the water content in hydrated Na 0.67 MnO 2 is ~0.45 mol per chemical formula unit (Supplementary Table 1 ), it is therefore reasonable to conclude that the C atoms in the bulk of the hydrated samples are negligible. Furthermore, the cross-sectional TOF-SIMS chemical mapping images of the tested secondary particles (Fig. 3c ) show that the intensity of C-related species (e.g. C 2 HO − , NaC 2 O 2 − , C − ) is much lower than OH − and Mn-based ions and the remaining carbonate trace is mainly distributed on the surface rather than the bulk of the particles. This fact coincides well with the depth profile results in Fig. 3b and Supplementary Fig. 9 . Therefore, the function of CO 2 is to increase the acidity at the particle’s surface and accelerate the Na + loss rather than insert into the bulk of the Na x TmO 2 phases. Fig. 3: TOF-SIMS results of the hydrated Na 0.67 MnO 2 sample. a the comparison of FTIR spectra of the hydrated Na 0.67 MnO 2 and hydrated Na 0.67 MnO 2 after the scavenging process, indicating that after scavenging, most of the sodium (bi)carbonate impurities was removed. b TOP-SIMS spectra of OH − , MnO − , MnO 2 − , and C 2 HO − secondary ion fragments over 500 s Cs + sputtering along the depth profile of the sample after scavenging processes. c TOF-SIMS chemical mapping of the hydrated Na 0.67 MnO 2 after the scavenging process, showing the distribution of OH − , MnO 2 − , MnO − , C 2 HO − , NaC 2 O 2 − , and C − secondary ions. Full size image The critical sodium contents ( n c ) for hydration Although Na 0.67 Ni 0.33 Mn 0.67 O 2 has been reported to be one of the most air-stable P2-Na x TmO 2 oxides, the chemical change is observed in the EDS mapping as demonstrated in Fig. 2i . Furthermore, as shown in Fig. 4a , with longer exposure time, the intensity of the NaHCO 3 diffraction peaks increases while the (002) diffraction peak shifts to lower 2-theta (Supplementary Fig. 10 ), suggesting the gradual extraction of Na + from Na 0.67 Ni 0.33 Mn 0.67 O 2 during exposure. To validate the identification of NaHCO 3 , the pristine and exposed Na 0.67 Ni 0.33 Mn 0.67 O 2 samples are further scrutinized by FTIR. As shown in Supplementary Fig. 11 , the characteristic peaks located at 600-2000 cm −1 in the FTIR spectrum of the exposed Na 0.67 Ni 0.33 Mn 0.67 O 2 in RH 93% + CO 2 fit well with that of NaHCO 3 . The absence of the O–H stretching signal between ~2500 and 3500 cm −1 suggests that no H 2 O intercalates into the sodium layers of Na 0.67 Ni 0.33 Mn 0.67 O 2 , which is highly consistent with the XRD results. In addition, as shown in Fig. 4b and Supplementary Fig. 12 , the 23 Na MAS NMR signal of Na 0.67 Ni 0.33 Mn 0.67 O 2 shifts to the upper field by 47 ppm, corresponding to the expansion of c parameter (Supplementary Fig. 10 ). It is worth noting that the intensity of 23 Na{ 1 H} REDOR signal for the exposed Na 0.67 Ni 0.33 Mn 0.67 O 2 sample decreases with 1 H irradiation as a function of the spin-echo time, as compared to that without 1 H irradiation. This result confirms that H + ions are in close proximity to the sodium atoms in the structure of the exposed Na 0.67 Ni 0.33 Mn 0.67 O 2 sample. Thus, it is more likely that the H ions replace those lost Na + , indicative of the Na + /H + exchange mechanism. Moreover, given that the exposed electrodes usually exhibit improved open circuit potential [26] , another charge compensation mechanism, i.e. the oxidation of transition metal ions by O 2 has been also proposed [5] . To validate which mechanism dominates the Na + loss process, X-ray absorption spectroscopy (XAS) was carried out. According to the previous results [8] , [20] , [49] , during the first charge process of Na 0.67 Ni 0.33 Mn 0.67 O 2 electrode within 2.0–4.4 V (vs. Na + /Na), Mn 4+ ions remain stable and the oxidation/reduction of Ni ions compensates the electrochemical extraction/insertion of Na + . As shown in Supplementary Fig. 13a , both position and shape of the Ni K-edge remain unchanged, indicating that the valence state of Ni ions in the exposed Na 0.67 Ni 0.33 Mn 0.67 O 2 is nearly the same as in the pristine sample. The valence state of Mn ions in pristine and hydrated Na 0.67 MnO 2 samples has been also investigated by XAS. The pre-edge peak and main edge of Mn K-edge XAS correspond to 1 s → 3 d and 1 s → 4 p transitions, respectively. However, the structural changes during hydration (Supplementary Fig. 13b ) severely complicate the chemical shift of the main edge such that it becomes difficult to determine the valence state of Mn ions. Thus the pre-edge region could provide more reliable valent-state information [50] . As can be seen from Supplementary Fig. 13b , the splitting and intensity of pre-edge peaks of Mn ions are similar for all of the pristine, partially hydrated and totally hydrated samples, indicating that the changes of the valence state of Mn ions are negligible during hydration. The XAS results suggest that Na + /H + exchange might be the main reaction that compensates for the extracted Na + in the moisture-exposed Na x TmO 2 . To confirm this conclusion, we stored the Na 0.67 MnO 2 sample in three different atmospheres for 3 days, e.g. O 2 , RH 93% + CO 2 with the presence of O 2 , and RH 93% + CO 2 without O 2 . The XRD patterns in Fig. 2a and Supplementary Fig. 13c suggest that O 2 makes smaller difference than both CO 2 and water to the structural changes of Na x TmO 2 . Fig. 4: The structural and chemical evolution mechanisms upon air-exposure. a The XRD evolutions of Na 0.67 Ni 0.33 Mn 0.67 O 2 powder exposed at RH 93% + CO 2 atmosphere for different times (MgO was used as internal indicator). b 23 Na{ 1 H} REDOR-dephased 23 Na MAS NMR spectra (MAS rate: 25 kHz) and c The XRD patterns of exposed Na x Ni 0.33 Mn 0.67 O 2 electrodes with various Na + content x. d The FTIR spectra of Na 0.67 MnO 2 samples with various hydration degrees. e The structure model of single layer Na + loss structure for calculating hydration energies. f The calculated hydration energies for Na x MnO 2 at various sodium contents x. Full size image To gain deeper insight into the structural/chemical transformation mechanisms of P2-Na x TmO 2 materials upon air-exposure, a series of Na x Ni 0.33 Mn 0.67 O 2 electrodes with different Na + contents were prepared by extracting Na + electrochemically, and then exposed at RH 93% + CO 2 atmosphere for 3 days. As shown in Fig. 4c , the hydration phase is absent at Na x Ni 0.33 Mn 2/3 O 2 electrodes within sodium contents of 0.67 ≤ x ≤ 0.44. In x = 0.38, the diffraction peaks of the hydration phase appear and its intensity increases with the further decrease of Na + contents. This result implies that hydration highly depend on the Na + contents. Specifically, if the sodium content x is lower than a critical sodium content n c (0.38–0.44 for Na x Ni 0.33 Mn 2/3 O 2 electrode), P2-Na x TmO 2 materials are vulnerable for hydration and vice versa. The correlation between hydration degree and sodium contents x is also observed in Na x MnO 2 compounds. As representatively shown in Fig. 4d , the intensity of NaHCO 3 absorption peaks are positively associated with the hydration degrees of Na 0.67 MnO 2 sample. The density function theory (DFT) calculation was carried out to further understand the critical sodium content n c . As shown in Fig. 4e and Supplementary Fig. 13d , two different sodium extraction models of single layer and double layer were considered, which correspond to the staging and random sodium extraction mechanisms, respectively [15] . The energy difference between P2-Na x TmO 2 with and without water molecules is defined as hydration energy. DFT calculation results in Fig. 4f show that when x > 0.52, the hydration energy of Na x MnO 2 is higher than 0 eV, suggesting that water molecules cannot get inserted into the material. When the sodium content is lower than 0.52, the hydration energy is lower than 0 eV, thus the hydrated structure is more stable than the un-hydrated structure. The foregoing energy analysis provides a chemical basis for understanding the sodium-content-dependent property in the hydration of Na x MnO 2 samples. Due to the low formation energy, the layered Na 0.67 TmO 2 oxides will lose Na + spontaneously once in contact with moist air. When the sodium contents are lower than n c , there is a strong repulsion between adjacent oxide layers (TmO 2 ) of P2-Na x TmO 2 oxides, and the insertion of H 2 O could lower the energy of Na 0.67-x-z H x TmO 2 (x and z correspond to the Na + loss that compensated by Na + /H + exchange and O 2 oxidation, respectively) due to the shielding effect of the water molecule and the expansion of sodium layer spacings. The above results also proved and interpreted the fact that hydration takes place after the extraction of Na + during air-exposure. Based on these results and analyses, the structural and chemical transformations of exposed P2-Na 0.67 TmO 2 to different ambient atmospheres are summarized in Eqs. ( 1 – 4 ). In the atmosphere without CO 2 : 
    x ·H_2O + Na_0.67TmO_2 = Na_0.67 - xH_xTmO_2 + x ·NaOH
 (1) In the atmosphere with scarce CO 2 : 
    x ·CO_2 + x ·H_2O + 2 ·Na_0.67TmO_2 =   2 ·Na_0.67 - xH_xTmO_2 
     	+ x ·Na_2CO_3
 (2) In the atmosphere with abundant CO 2 : 
    x ·CO_2 + x ·H_2O + Na_0.67TmO_2 = Na_0.67 - xH_xTmO_2 
     	+ x ·NaHCO_3
 (3) If the sodium content in the electrode is lower than n c : 
    Na_0.67 - xH_xTmO_2 + y ·H_2O = [ Na_0.67 - xH_x(H_2O)_y]TmO_2
 (4) It should be emphasized that although Tm oxidation is not included in the proposed charge-compensation mechanisms due to lacking of direct spectroscopic evidences, there is still a high possibility that a minority of charge is compensated by the valence change of Tm ions. In the near future, more techniques, especially the state-of-the-art s-XAS characterizations are expected to obtain a deeper understanding of the charge-compensation mechanisms of Na + extraction in moisture-exposed Na x TmO 2 . The influence of structural changes on the electrochemical performances of P2-Na x TmO 2 In this section, we carefully investigate the influences of the above structural and chemical changes on the electrochemical performances of Na 0.67 MnO 2 and Na 0.67 Ni 0.33 Mn 2/3 O 2 electrodes. As shown in Fig. 5a , the pristine Na 0.67 MnO 2 shows a high initial discharge capacity of 176 mAh g −1 at the current density of 12 mA g −1 within 2.0–4.4 V. After 50 cycles, 66 % of the initial capacity was retained, which coincides well with the previous results [10] , [23] . For the hydrated Na 0.67 MnO 2 electrode, the reversible capacity is negligible at the initial cycles. In the 9 th cycle, although the discharge capacity increased to ~150 mAh g −1 , abnormal electrochemistry, such as long charging plateaus, large voltage hysteresis and low coulombic efficiency are also observed. These deviant electrochemical performances indicate that the large amount of H 2 O in the hydrated electrode has a pernicious influence on the organic-electrolyte based batteries. Fig. 5: Electrochemical performances of air-exposed Na 0.67 MnO 2 and Na 0.67 Ni 0.33 Mn 0.67 O 2 . a The cycling performance of pristine Na 0.67 MnO 2 , the inset shows the charge-discharge curve at the 2nd cycle. b The charge-discharge curves and cycling stability of totally hydrated Na 0.67 MnO 2 sample. c – f The electrochemical performances within the voltage range of 2.0–4.0 V of three Na 0.67 Ni 0.33 Mn 0.67 O 2 samples (pristine Na 0.67 Ni 0.33 Mn 0.67 O 2 , Na 0.67 Ni 0.33 Mn 0.67 O 2 samples immersed in water for 20 days and exposed in RH 93% + CO 2 for 3 days). c The initial charge-discharge curves at 12 mA g −1 . d The cycling stability of the three samples at 120 mA g −1 (after two formation cycles at 12 mA g −1 ). e The comparison of the impedance responses at the 1st and 100th cycles with frequency varied from 100 kHz to 10 mHz. f The rate capability of three samples at the voltage range of 2.0–4.0 V. Full size image The electrochemical performances of pristine Na 0.67 Ni 0.33 Mn 0.67 O 2 , Na 0.67 Ni 0.33 Mn 0.67 O 2 exposed in RH 93% + CO 2 for 3 days (denoted as exposed-Na 0.67 Ni 0.33 Mn 0.67 O 2 ), and Na 0.67 Ni 0.33 Mn 0.67 O 2 immersed in water for 20 days (denoted as immersed-Na 0.67 Ni 0.33 Mn 0.67 O 2 ) are presented in Fig. 5c–f . As shown in Fig. 5c , the pristine Na 0.67 Ni 0.33 Mn 0.67 O 2 , exposed-Na 0.67 Ni 0.33 Mn 0.67 O 2 , and immersed-Na 0.67 Ni 0.33 Mn 0.67 O 2 samples have very similar initial charge-discharge curves, suggesting that their structure and redox center are nearly identical [8] . However, the initial charge capacities of the exposed-Na 0.67 Ni 0.33 Mn 0.67 O 2 (70 mAh g −1 ) and immersed-Na 0.67 Ni 0.33 Mn 0.67 O 2 (77 mAh g −1 ) are lower than that of the pristine Na 0.67 Ni 0.33 Mn 0.67 O 2 (85 mAh g −1 ), further confirming the loss of Na + ions during the exposure and immersing processes. Fig. 5d compares the cycling stability of the three electrodes. It can be observed that the exposed-Na 0.67 Ni 0.33 Mn 0.67 O 2 exhibits much lower coulombic efficiency than the pristine Na 0.67 Ni 0.33 Mn 0.67 O 2 , due to the influence of the sodium bicarbonate on the surface of exposed-Na 0.67 Ni 0.33 Mn 0.67 O 2 particles. At the voltage range of 2.0–4.0 V, the pristine Na 0.67 Ni 0.33 Mn 0.67 O 2 material shows no evidence of capacity degradation after 100 cycles. In contrast, the immersed-Na 0.67 Ni 0.33 Mn 0.67 O 2 and exposed-Na 0.67 Ni 0.33 Mn 0.67 O 2 samples decay fast in capacity, and retain low discharge capacity of 56 and 53 mAh g −1 , corresponding to the capacity retention of 74% and 70%, respectively. To get more insight into the degradation mechanisms, the electrochemical impedance spectra (EIS) have been employed to study the resistance changes. The interface and charge-transfer resistances were estimated based on the equivalent circuit in Supplementary Fig. 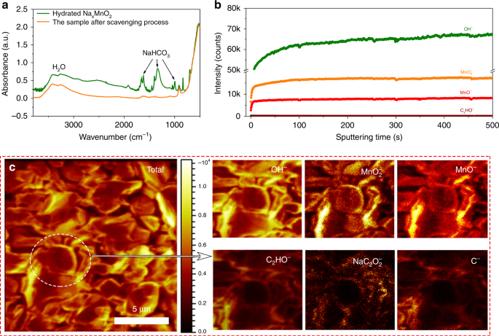Fig. 3: TOF-SIMS results of the hydrated Na0.67MnO2sample. athe comparison of FTIR spectra of the hydrated Na0.67MnO2and hydrated Na0.67MnO2after the scavenging process, indicating that after scavenging, most of the sodium (bi)carbonate impurities was removed.bTOP-SIMS spectra of OH−, MnO−, MnO2−, and C2HO−secondary ion fragments over 500 s Cs+sputtering along the depth profile of the sample after scavenging processes.cTOF-SIMS chemical mapping of the hydrated Na0.67MnO2after the scavenging process, showing the distribution of OH−, MnO2−, MnO−, C2HO−, NaC2O2−, and C−secondary ions. 14 and summarized in Supplementary Table 3 . In the first cycle, the electrode resistance of the three samples is quite similar (the inset in Fig. 5e ). After 100 cycles, the rapid increase of the surface resistance (R SEI ) and charge transfer resistance (R C, CT ) for the exposed-Na 0.67 Ni 0.33 Mn 0.67 O 2 and immersed-Na 0.67 Ni 0.33 Mn 0.67 O 2 (Fig. 5e ) samples indicates that the decomposition layer on the surface and the proton ions in the structure accelerate the depletion of the electrolyte thus blocking the diffusion of Na + ions. The comparison of rate capabilities shows a similar trend of cycling stability. As shown in Fig. 5f , the pristine Na 0.67 Ni 0.33 Mn 0.67 O 2 electrode exhibits higher capacities than the immersed and exposed samples at all rates. The above electrochemical results demonstrate that exposure to moist air and immersion in water cause undesired structural changes and result in deteriorated electrochemical performances of P2-Na x TmO 2 samples. The structural transformation of hydrated phases upon calcination in air We have concluded that the sodium extraction (mainly compensated by Na + /H + exchange) and H 2 O insertion are two continuous structural transition processes during the exposure of P2-Na x TmO 2 samples, which usually impair their intrinsic electrochemical performances. The following questions need to be clarified: (i) whether or not these exposed samples can be recovered to their original structure and how, and (ii) what is the stoichiometry of hydrated phases (birnessite)? Therefore, in this section, the structural transitions of hydrated samples at the temperature range of 25–570 °C were investigated by in situ variable-temperature XRD technique. As shown in Fig. 6 , five different stages can be observed in the in situ variable-temperature XRD pattern of the hydrated Na 0.67 MnO 2 . The mass loss at stage a (25–130 °C) is ~15.1%, which includes decomposition of NaHCO 3 [51] and extraction of water. At this stage, the hydration structure is well maintained. From stage a to stage b , the hydrated phase is most probably transformed into a protonated phase (Supplementary Fig. 15 and Note 5 ) by two-phase reaction mechanisms at ~130 °C. The crystallinity of the Na 0.67-x-z MnO 2 phase at stage c (217–297 °C) is much lower than stage b , which might be resulted from the loss of protons. In addition, the sodium carbonate begins to decompose and results in the mass loss in stage c . With further increase in temperature, the crystallinity of Na 0.67-x-z MnO 2 increases, as shown in stage d . It should be pointed out that the decomposition temperature of Na 2 CO 3 is lower than 800 °C due to the small sizes of the Na 2 CO 3 particles (Fig. 2 and Supplementary Fig. 5 ) and the catalytic effect of transition metal oxides on reducing the energy requirement of Na 2 CO 3 decomposition [52] . When the temperature is higher than 483 °C, the (100) and (103) peaks (at ~35° and ~43°, respectively) of the P2 phase emerge gradually, indicating the P2-Na 0.67 MnO 2 phase gradually recovers at stage e . 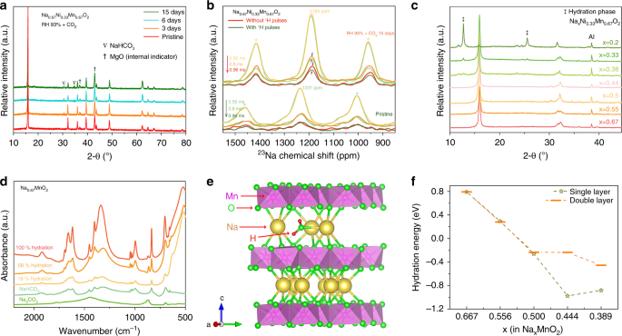Fig. 4: The structural and chemical evolution mechanisms upon air-exposure. aThe XRD evolutions of Na0.67Ni0.33Mn0.67O2powder exposed at RH 93% + CO2atmosphere for different times (MgO was used as internal indicator).b23Na{1H} REDOR-dephased23Na MAS NMR spectra (MAS rate: 25 kHz) andcThe XRD patterns of exposed NaxNi0.33Mn0.67O2electrodes with various Na+content x.dThe FTIR spectra of Na0.67MnO2samples with various hydration degrees.eThe structure model of single layer Na+loss structure for calculating hydration energies.fThe calculated hydration energies for NaxMnO2at various sodium contents x. However, the mass loss of 0.45% during 130–217 °C corresponds to x = 0.61 in Na 0.67-x-z H x MnO 2 , exceeding the amount of lost Na + ions ( x + z ≈ 0.39, Supplementary Table 4 ), suggesting that the decomposition of Na 2 CO 3 begins at stage b (130–217 °C). In conclusion, with the increase of temperature, the hydrated Na 0.67 MnO 2 sample undergoes dehydration and NaHCO 3 decomposition (70–130 °C), deprotonation (130–217 °C), Na 2 CO 3 decomposition (>130 °C) and the recrystallization of P2 phase (>483 °C) process. In our recent work [23] , we demonstrate that Na 0.67 Zn 0.1 Mn 0.67 O 2 is a promising Na-ion battery cathode with outstanding cycling stability and better air-stability than Na 0.67 MnO 2 . Therefore, we also performed the in situ variable-temperature XRD of totally hydrated Na 0.67 Zn 0.1 Mn 0.9 O 2 powder. Obviously, the structural transformation of the hydrated Na 0.67 Zn 0.1 Mn 0.9 O 2 in Supplementary Fig. 16 is different from that of the hydrated Na 0.67 MnO 2 . From the hydration phase (stage a ) to the protonated phase (stage b ), the combined mechanism of two-phase and solid-solution reactions can be recognized. Moreover, the temperature range of deprotonation of the hydrated Na 0.67 Zn 0.1 Mn 0.9 O 2 sample is elusive and the temperature of the recrystallization of P2-type Na 0.67 Zn 0.1 Mn 0.9 O 2 phase (376 °C) is lower than that of Na 0.67 MnO 2 (483 °C). The above results indicate that if the Na 0.67 TmO 2 samples undergo sodium-loss and further hydration processes upon air-exposure, high-temperature annealing can be used to recover their original structures (the results of verification test are shown in Supplementary Fig. 17 and Note 6 ). Although the detailed structural transformation mechanisms during annealing are highly dependent on the stoichiometry of the exposed Na 0.67 TmO 2 , the general structural/chemical evolution processes are concluded in Eqs. ( 5 – 7 ) (Supplementary Note 7 and 8 ). Fig. 6: Temperature-resolved in situ XRD of the totally hydrated Na 0.67 MnO 2 . The temperature ranges from 25 to 570 °C. The TGA curves are shown at the left. Hydrated and P2 phases are labeled with “‡” and “†”, respectively. Full size image 30–130 °C: 
    2x ·NaHCO_3 = x ·Na_2CO_3 + x ·H_2O + x ·CO_2
 (5) 
    [Na_0.67 - xH_x(H_2O)_y]TmO_2 = y ·H_2O + [Na_0.67 - xH_x]TmO_2
 (6) 130–900 °C: 
    2 ·[ Na_0.67 - xH_x]TmO_2 + x ·Na_2CO_3 =   x ·H_2O + x ·CO_2 
     + 2 ·Na_0.67TmO_2
 (7) According to the structural/chemical evolution processes revealed by the above in situ XRD patterns, the chemical formulas of several hydrated Na 0.67 TmO 2 materials, including Na 0.67 MnO 2 , Na 0.67 Al 0.1 Mn 0.9 O 2 , Na 0.67 Cu 0.1 Mn 0.9 O 2 , Na 0.67 Zn 0.1 Mn 0.9 O 2 , and Na 0.67 Zn 0.2 Mn 0.8 O 2 , are identified based on the TGA analysis (see detailed information in Supplementary Figs. 18 and 19 , Table 4 , Supplementary Eqs. ( 1 – 8) , and Supplementary Note 8 ). ICP-AES analyses in Supplementary Table 4 are in good agreement with the chemical formulas of hydration phases. The results suggest that the contents of inserted H 2 O vary greatly from ~0.1 to 0.45 depending on the stoichiometry of pristine materials. The comprehensive structural/chemical evolution mechanisms upon air-exposure Based on our analysis above, we summarize the structural and chemical transitions of the P2-Na 0.67 TmO 2 components upon air exposure in Fig. 7a . At the initial stage, because of the low formation energy of layered Na 0.67 TmO 2 oxides, the sodium ions are lost from the bulk and form amorphous Na 2 CO 3 /NaHCO 3 layer on the surface of particles or even Na 2 CO 3 /NaHCO 3 crystals with charge-compensation mechanism of Na + /H + exchange. The formation energy increases with the extraction of Na + ions and finally the P2-Na x TmO 2 oxides are stable at the sodium content of 0.67-x-z in a specific environment. If the remaining sodium content 0.67-x-z is lower than the critical sodium content n c , the water molecules go into the sodium layers and form the hydration phases. Considering the full decomposition of generated sodium salts and the recrystallization of the degraded structures, once the Na 0.67 TmO 2 is protonated or hydrated, high-temperature calcination is needed to recover the hydrated forms back to the original structure. In addition to the above structural transitions, the outer layer of Na x TmO 2 particles decomposes into transition-metal oxides/hydroxides when exposed to air or immersed in water. As shown in Supplementary Fig. 20 , after exposing Na 0.67 Cu 0.33 Mn 0.67 O 2 at RH 93% + CO 2 for 6 days, the Cu 2 O and NaHCO 3 impurities can be observed in the XRD pattern, indicating that degradation is more or less an inevitable process at the surface of exposed Na 0.67 TmO 2 compounds. Manthiram’s group also reported that the Ni-rich layered sodium oxide transforms into NiO and Na 2 CO 3 in the surface [26] . In brief, the structural and chemical transitions coexist, rather than a single protonation/Tm-oxidation, hydration, and degradation mechanism. Fig. 7: Reaction pathways and evaluation rule. a Proposed reaction pathways for the moisture-exposed Na 0.67 TmO 2 materials. b The comparison of the main redox couples in layered sodium transition metal oxides. Full size image Evaluating the air-stability of Na x TmO 2 electrodes The choice and evaluation of air-stable Na x TmO 2 electrodes have attracted enormous attention. It has been widely accepted that the Ni/Mn superlattice prevents the intercalation of H 2 O since P2-Na 0.67 Ni 0.33 Mn 0.67 O 2 was found to be resistant to hydration in moisture [27] . However, our results demonstrate that Na 0.67 Ni 0.33 Mn 0.67 O 2 is not as stable in moist air as it was expected, while other reported air-stable electrodes, such as Na 0.78 Cu 0.27 Zn 0.06 Mn 0.67 O 2 [32] , Na 0.67 Ni 0.22 Cu 0.11 Ti 0.11 Mn 0.56 O 2 [35] and Na 7/9 Cu 2/9 Fe 1/9 Mn 2/3 O 2 [53] do not have superlattice ordering in Tm layers. Therefore, the crucial factors, as well as the evaluation principles related to the air-stability of Na x TmO 2 electrodes, have yet to be re-explored. Therefore, we compared the air-stability of five layered oxides with different Mn valence-state and redox potential, e.g. Na 0.67 MnO 2 , Na 0.67 Al 0.1 Mn 0.9 O 2 , Na 0.67 Zn 0.1 Mn 0.9 O 2 , Na 0.67 Zn 0.2 Mn 0.8 O 2 and Na 0.67 Ni 0.33 Mn 0.66 O 2 , at the atmosphere of dry CO 2 , RH 18%, RH 15% + CO 2 , and RH 93% + CO 2 . The XRD patterns and ICP-AES results of these pristine oxides are presented in Supplementary Fig. 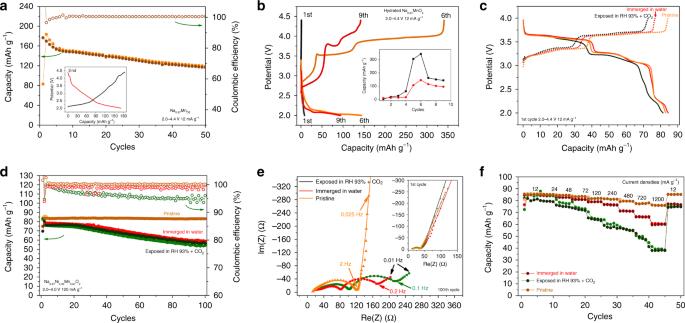Fig. 5: Electrochemical performances of air-exposed Na0.67MnO2and Na0.67Ni0.33Mn0.67O2. aThe cycling performance of pristine Na0.67MnO2, the inset shows the charge-discharge curve at the 2nd cycle.bThe charge-discharge curves and cycling stability of totally hydrated Na0.67MnO2sample.c–fThe electrochemical performances within the voltage range of 2.0–4.0 V of three Na0.67Ni0.33Mn0.67O2samples (pristine Na0.67Ni0.33Mn0.67O2, Na0.67Ni0.33Mn0.67O2samples immersed in water for 20 days and exposed in RH 93% + CO2for 3 days).cThe initial charge-discharge curves at 12 mA g−1.dThe cycling stability of the three samples at 120 mA g−1(after two formation cycles at 12 mA g−1).eThe comparison of the impedance responses at the 1st and 100th cycles with frequency varied from 100 kHz to 10 mHz.fThe rate capability of three samples at the voltage range of 2.0–4.0 V. 21 and Table 5 , respectively. In addition, the XRD patterns and the corresponding quantification of the hydration extents of the exposed samples are shown in Supplementary Fig. 22 . According to the refinement results in Supplementary Fig. 22e , it is confirmed once again that more structural and chemical changes of Na 0.67 TmO 2 occur with the increase of relative humidity and the presence of CO 2 . Moreover, it can be clearly observed that the air-stability of these investigated layered oxides follows the order of Na 0.67 Ni 2+ 0.33 Mn 4+ 0.67 O 2 > Na 0.67 Zn 2+ 0.2 Mn 3.66+ 0.8 O 2 > Na 0.67 Zn 2+ 0.1 Mn 3.47+ 0.9 O 2 > Na 0.67 Al 3+ 0.1 Mn 3.37+ 0.9 O 2 > Na 0.67 Mn 3.33+ O 2 , suggesting that the air-stability is closely related to the valence state of Mn ions or the redox potential of the initial charge process (Supplementary Fig. 23 ). 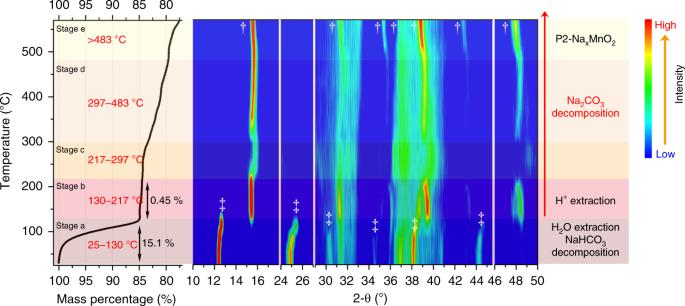Fig. 6: Temperature-resolved in situ XRD of the totally hydrated Na0.67MnO2. The temperature ranges from 25 to 570 °C. The TGA curves are shown at the left. Hydrated and P2 phases are labeled with “‡” and “†”, respectively. 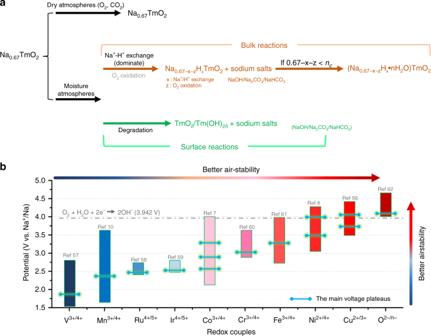Fig. 7: Reaction pathways and evaluation rule. aProposed reaction pathways for the moisture-exposed Na0.67TmO2materials.bThe comparison of the main redox couples in layered sodium transition metal oxides. To confirm this hypothesis, several electrodes were prepared and exposed to the atmosphere of RH 93% + CO 2 . As shown in Supplementary Fig. 24 , although the valence state of Mn ions in Na 0.67 Co 3+ 0.67 Mn 4+ 0.33 O 2 , Na 0.67 Ni 2+ 0.17 Co 3+ 0.33 Mn 4+ 0.50 O 2 and Na 0.67 Ni 2+ 0.17 Fe 3+ 0.33 Mn 4+ 0.50 O 2 electrodes are Mn 4+ , all of these samples are hydrated after three days’ exposure in the atmosphere of RH 93% + CO 2 , indicating that the valence state of Mn ions is not the key parameter for the air-stability property. Therefore, Na 0.67 Li 0.20 Mn 0.80 O 2 [54] , Na 0.67 Mg 0.28 Mn 0.72 O 2 [55] and Na 0.67 Cu 0.33 Mn 0.67 O 2 [56] samples that have high initial charging potential were prepared and exposed to the same atmosphere. As shown in Supplementary Fig. 20 and 25 , after the exposure for 3 or 6 days, no hydration peaks can be recognized, indicating that the Na 0.67 TmO 2 components with higher redox potential in the first cycles exhibit better air-stability. Generally, for a Na 0.67 TmO 2 material with higher electrochemical redox potential (equilibrium potential), it is more difficult to extract Na + from the lattice chemically. Therefore, the potential of redox couples could be considered as one of the key principles to evaluate the air-stability of Na 0.67 TmO 2 electrodes. Based on the above conclusion, we summarize the main redox couples in P2-Na x TmO 2 electrodes (Fig. 7b ), including V 3+/4+ [57] , Mn 3+/4+ [10] , Ru 4+/5+ [58] , Ir 4+/5+ [59] , Co 3+/4+ [7] , Cr 3+/4+ [60] , Fe 3+/4+ [61] , Ni 2+/4+ [8] , Cu 2+/3+ [56] , and O 2-/n- [62] . The result suggests that the electrodes with redox couples of Ni 2+/4+ , Cu 2+/3+ , and O 2−/n− show much better air-stability than that with the redox couples of V 3+/4+ , Mn 3+/4+ , Co 3+/4+ , Fe 3+/4+ , etc., which is in good agreement with the previous articles [5] , [32] , [34] , [35] , [63] . Besides chemical compositions, the crystallinity of Na 0.67 TmO 2 also makes a great difference to their air-stability. Supplementary Fig. 26a,b show the weight loss and XRD evolutions during the preparation process of Na 0.67 MnO 2 , respectively. When the temperature increases to 480 °C, Na 2 CO 3 begins to decompose and the β-MnO 2 (JCPDF: 72–1984) starts to transform into the layered Na 0.67 MnO 2 . The XRD peaks of β-MnO 2 disappear at ~540 °C and all of the Na 2 CO 3 is decomposed at ~ 640 °C. We compared the air-stability of the Na 0.67 MnO 2 samples at 640 °C, 900 °C, and the sample calcinated at 900 °C for 900 min, which exhibit increased crystallinity (Supplementary Fig. 26b ). As shown in Supplementary Fig. 26c , after being exposed in RH 18% atmosphere for 3 days, the hydration degree follows the order of 640 °C > 900 °C > 900 °C 900 min samples, and clearly indicates that the samples with higher degree of crystallinity exhibit better air-stability. In summary, a comprehensive investigation of the structural and chemical transformations of P2-Na x TmO 2 in different ambient atmospheres has been carried out. Using advanced technique characterizations and systematic investigation, we clarified and rationalized these intertwined reaction processes and their determining factors. For example, the critical roles of relative humidity and CO 2 in the air-stability of P2-Na 0.67 TmO 2 , the extraction of Na + ions from Na 0.67 Ni 0.33 Mn 0.67 O 2 when exposed to moist air or emerged in water, the influence of moisture-exposure on the electrochemical performances of Na x TmO 2 , the precise quantification of water contents in hydrated phases, and the significance of crystallinity on the air-stability of Na x TmO 2 , etc. Furthermore, based on the detailed mechanisms, including the Na extraction at the initial stage of moisture-exposure, the dominate Na + /H + exchange charge-compensation mechanism, and the critical sodium content ( n c ), we proposed a general and in-depth picture on the chemical/structural evolutions of P2-Na x TmO 2 during moisture-exposure. In addition, by extending the study to a variety of layered sodium-based oxides (Na 0.67 M x Mn 1-x O 2 , with M = Ni, Zn, Fe, Al, Co, Li, Mg, Cu, etc.) we have also demonstrated that the redox potential properties in the first charge process could be used as an empirical rule for evaluating the air-stability of Na x TmO 2 electrodes. Our results provide significant new clues for the design, synthesis, storage, and application of layered sodium cathodes, as well as other alkali-metal transition metal oxides. Preparation of layered materials The pristine Na x TmO 2 cathodes have been synthesized by high-temperature solid-state reactions [12] , [23] . Stoichiometric amounts of raw materials, e.g. MnO 2 (99.95%, Aladdin), ZnO (99.99%, Aladdin), NiO (99.99%, Aladdin), Al 2 O 3 (99.99%, Aladdin), TiO 2 (99.8%, Aladdin), CuO (99.9%, Aladdin), Li 2 CO 3 (99.99%, Aladdin), and Na 2 CO 3 (99.99%, Aladdin) were ball-milled with acetone solvent for 3.5 h at 500 rpm. Then dried at 120 °C overnight, pressed into pellets and heated at 900 °C for 15 h in air. After slowly cooled to 150 °C in the furnace, the pellets were transferred to an Ar-filled glove box immediately, ground and kept the final products in the Ar-filled glove box. Hydration tests The saturated salt solutions could produce stable relative humidity in a closed system at a certain temperature [64] , [65] . To study the effect of different ambient atmospheres on the structural and chemical stability of Na x TmO 2 , the prepared Na 0.67 TmO 2 oxides are put in a centrifuge tube and then aged on an airtight container under four different storage conditions at the constant temperature of 40 °C. They are dry CO 2 , controlled humidity of RH 18% (without CO 2 ), RH 15% with CO 2 , and RH 93% with CO 2 . To maintain the ambience conditions of dry CO 2 , RH 15% with CO 2 and RH 93% with CO 2 , the dry silica gel, saturated aqueous LiCl and NaHCO 3 solutions are placed below the samples, respectively. After that, the containers are filled with CO 2 . The RH 18% (without CO 2 ) atmosphere was obtained by placing the saturated NaOH solution at the bottom of the container and then filled with dry O 2 . The accurate RH is determined by a hygrometer, whose accuracy is ±1%. The elemental compositions of pristine and exposed samples were confirmed by inductively coupled plasma-atomic emission spectrometry (ICP-AES) analysis (IRIS Intrepid II XSP, Thermo Electron). Before ICP-AES and Time-of-flight secondary ion mass spectroscopy (TOF-SIMS) testing, we applied a scavenging process to remove the Na 2 CO 3 /NaHCO 3 byproducts in the exposed samples. Specifically, the exposed samples were immersed and stirred in distilled water for 3 min, then centrifuged and dried at 80 °C overnight. Characterizations The X-ray diffraction (XRD) patterns were obtained on a Rigaku Ultima IV diffractometer by a Persee instrument with Cu Kα radiation ( λ = 1.5406 Å). The patterns were refined by the General Structure Analysis System (GSAS) software [44] . The morphologies of samples were characterized by scanning electron microscopy (SEM, Hitachi S-4800). The EDS elemental mapping experiments were conducted using FEI Talos-F200s TEM instrument. The 23 Na ss-NMR experiments were acquired on a Bruker AVANCE III 400 MHz spectrometer using a double resonance 1.3 mm MAS probe spinning at frequencies of up to 55 kHz with a Hahn-echo pulse sequence (i.e. 90 o pulse – τ – 180 o pulse – τ, where τ is set to a multiple of rotor periods). The 90 o pulse length of 1.2 μs and a recycle delay of 2 ms were used. The 23 Na shifts were referenced to 1 M NaCl aqueous solution (0 ppm). For 1 H, the 2.5 mm MAS probe was used spinning at 25 kHz to record the 1 H spectra with the rotor-synchronized Hahn Echo sequence and a cycle delay of 2 s and a 90 o pulse length of 4 μs. No window functions were added and the chemical shift of 1 H was referenced against adamantane (1.87 ppm). By using 2.5 mm MAS probe with a MAS rate of 25 kHz, the rotational echo double resonance (REDOR) NMR sequence (i.e. the rotor-synchronized Hahn echo is applied on 23 Na, during τ periods the 23 Na- 1 H dipolar coupling is recovered by 180 o 1 H pulses) is applied to confirm the presence of H + in the exposed materials. Geometry-independent information about the 23 Na- 1 H dipole couplings can be conveniently obtained from the plot of signal attenuation (1-scale) versus the dipolar evolution time (2tau). In all MAS NMR measurements, the variable temperature (VT) gas temperature was set to 315 K. The in situ XRD experiments were performed in air and on a BrukerD8 Discover diffractometer equipped with a Cu Kα radiation. Infrared spectra were recorded on a Nicolet is50 FT-IR (Thermo Fisher Scientific Inc., Madison, USA) spectrometer. X-ray absorption spectroscopy (XAS) data were acquired in the transmission mode at the BL14W1 beamline of the Shanghai synchrotron radiation facility (SSRF) at room temperature, and the incident beam was monochromatized by a Si (111) double-crystal monochromator. TOF-SIMS were performed on a TOF-SIMS5 spectrometer (ION TOF GmbH). The depth profiling and high-resolution mapping were conducted at the high current mode and burst alignment mode, respectively, with a pulsed Bi 1 + ion beam (30 keV). The sputtering was conducted by a 500 eV Cs + ion beam with the area of 100 μm × 100 μm, and the analyzed areas for depth profiling and high-resolution mapping are typically 100 μm × 100 μm and 50 μm × 50 μm with the pixel of 128 × 128. Electrochemical tests The electrodes are composed of 80 wt% of active materials, 10 wt% of polyvinylidene fluoride (PVDF) and 10 wt% acetylene carbon black. The mass loading of active materials is 2.5–3 mg cm −1 . The cleaned aluminum foil was used as current collector. The electrochemical performances were tested in 2025 coin cells which assembled in an Ar-filled glove box, using 1 M NaPF 6 in Propylene carbonate (PC, 98 vol%) and Fluoroethylene carbonate (FEC, 2 vol%) as the electrolyte, Whatman glass fiber filter as the separator, and sodium metal as the counter electrode. The galvanostatic charge-discharge processes were conducted on multichannel battery tester (Neware, CT-4008-5V10mA-164). The electrochemical impedance spectroscopy (EIS) was conducted by a four-channel multifunctional electrochemical workstation (Versa STAT MC. America), at the cell voltage of 4.0 V and with the frequency range of 100 kHz to 0.01 Hz. DFT calculation The DFT calculations were performed on VASP (Vienna ab initio Simulation Package) [66] and the exchange-correlation interactions of electron were described with spin-polarized generalized gradient approximation (GGA) and parameterized by PBE formula [67] . The projector-augmented wave approach and GGA + U method were used to evaluate the electron-ion interactions and the localization of the d electrons of the TM ions, respectively [68] , [69] . The U value of Mn set to 3.9 eV and the wave functions were expended by plane wave with a kinetic energy cut-off of 520 eV. The Monkhorst–Pack scheme [70] was used for the integration in the irreducible Brillouin zone with a k-point mesh resolution of 2π × 0.025 Å −1 . The lattice parameters and atomic coordinates were fully relaxed, and the final forces on all atoms were <0.01 eV Å −1 . For the DFT calculations, a 3 × 3 × 1 supercell, which contains 12 Na, 36 O, and 18 Mn has been adopted. Sodium contents of x = 0.667, 0.556, 0.500, 0.444 and 0.389 in Na x MnO 2 correspond to 12, 10, 9, 8 and 7 Na ions in the supercell, and the number of different structures for each Na contents is \(C_{12}^0\) , \(C_{12}^2\) , \(C_{12}^3\) , \(C_{12}^4\) , and \(C_{12}^5\) , respectively. Therefore, 1574 kinds of structures should be considered based on the enumeration method. Such computation load is however too heavy to be carried out and 9 of them have been calculated. Specifically, we considered two different sodium extraction models for the five different Na contents. The number of calculated structures for x = 0.667, 0.556, 0.500, 0.444 and 0.389 in Na x MnO 2 are 1, 2, 2, 2, 2, respectively, as shown in Fig. 4f (page 11 in the manuscript). Moreover, the residual Na sites were chosen randomly and then one water molecule was put into an empty Na site also randomly.